Monolithic graphene oxide sheets with controllable composition Graphene oxide potentially has multiple applications and is typically prepared by solution-based chemical means. To date, the synthesis of a monolithic form of graphene oxide that is crucial to the precision assembly of graphene-based devices has not been achieved. Here we report the physical approach to produce monolithic graphene oxide sheets on copper foil using solid carbon, with tunable oxygen-to-carbon composition. Experimental and theoretical studies show that the copper foil provides an effective pathway for carbon diffusion, trapping the oxygen species dissolved in copper and enabling the formation of monolithic graphene oxide sheets. Unlike chemically derived graphene oxide, the as-synthesized graphene oxide sheets are electrically active, and the oxygen-to-carbon composition can be tuned during the synthesis process. As a result, the resulting graphene oxide sheets exhibit tunable bandgap energy and electronic properties. Our solution-free, physical approach may provide a path to a new class of monolithic, two-dimensional chemically modified carbon sheets. Graphene oxide (GO) is a material of great interest for its potential applications in nanoelectronics [1] , [2] , sensors [3] , energy storage devices [4] and light-emitting devices [5] , [6] . GO is an atomically thin sheet consisting of graphite that is decorated with oxygen (O)-containing functional groups, and it contains a mixture of sp 2 - and sp 3 -hybridized carbon (C) atoms bearing hydroxyl (C–OH) and epoxide (C–O–C) functional groups on the basal plane and carbonyl (C=O) and carboxyl (COOH) groups at the sheet edges [5] . Graphene in itself does not have a native oxide, and harsh chemical treatments are necessary to produce GO films [7] . GO is typically prepared by solution-based chemical means from micrometre-scale graphite flakes, and properties of GO-based devices depend on the preparation process used, which can yield a range of network morphologies of GO flakes [8] , [9] , [10] , [11] . Chemically derived GO is electrically insulating and must be reduced using chemical and/or thermal treatment to make it electrically active [12] , [13] . Although the chemical routes might be preferred for large-volume manufacturing, they can be less effective to offer paths towards precise device assembly, owing to the enormous interlayer van der Waals forces and hydrophilic nature of GO [11] . To date, the synthesis of monolithic GO sheets has not been achieved on any surface over a large area, which limits their usefulness in device applications based on graphene and its derivatives. Here we demonstrate that a monolithic form of GO sheets can be physically synthesized on a copper (Cu) surface at low temperatures (≤260 °C), with tunable oxygen-to-carbon (O/C) composition. In our approach, we build a graphene framework on the reverse side of a Cu foil at a Cu/substrate interface by exploiting the solid-state diffusion of C atoms across a diffusion couple composed of a C–Cu/substrate. A combined experimental and theoretical study shows that the Cu foil provides an effective pathway for C diffusion, trapping the O species dissolved in Cu and enabling the formation of monolithic GO sheets on its surface after an incubation time. In contrast to chemically derived GO [8] , [9] , [10] , [11] , the as-synthesized GO sheets are electrically active and the O/C composition in GO can be tuned during the synthesis process by controlling the O content in the Cu foil before the solid-state diffusion process. The resulting GO sheets exhibit tunable bandgap energy by varying the O/C composition, making them potentially useful for flexible and transparent semiconducting applications. The GO films show the ambipolar transfer characteristics in bottom-gate field-effect transistor (FET) architectures, and the electronic properties are found to correlate closely with the bandgap energy. These results suggest that monolithic, two-dimensional (2D) chemically modified C sheets with controllable composition can be prepared at low temperatures, which is highly desirable for graphene-based device production. 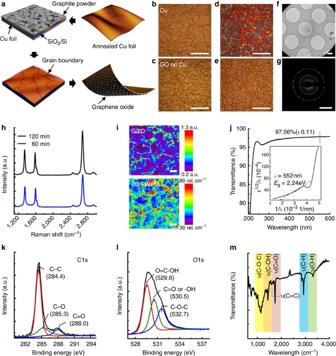Figure 1: Structural and optical characterization of monolithic GO sheets on Cu. (a) Schematic representation of the modified DAS process for obtaining monolithic GO sheets on the reverse side of a Cu foil. This process includes the elementary steps in the DAS process: the annealing of the Cu foil; the physical attachment of the Cu foil onto the substrate and the preparation of the C–Cu–substrate diffusion couple; heating of the assembly in ambient argon (below 260 °C) and the formation of monolithic GO sheets at the Cu/substrate interface; and the detachment of the Cu foils after removal of the solid C sources from the foil surface. (b–e) Optical microscopy images of annealed Cu foils (b,d) and GO-covered Cu foils (c,e) before (b,c) and after (d,e) oxidation in air at 200 °C for 120 min (scale bars, 150 μm). (f,g) A bright-field TEM image of the GO sheet (scale bar, 1 μm) (f) and its corresponding selected area electron diffraction pattern (scale bar, 5 nm−1). (g) Most micro-crystallites were polycrystalline. (h) Representative Raman spectra of GO that was grown on a Cu surface at 240 °C for 60 min (bottom) and 120 min (top), and then transferred onto SiO2(300 nm)/Si. (i) Raman map of the G/2D bands (top) and the FWHM of the 2D band (bottom) of GO that was grown on Cu at 240 °C for 60 min and then transferred onto SiO2(300 nm)/Si (scale bars, 10 μm). (j) Optical transmittance of GO that was grown on Cu at 240 °C for 120 min and then transferred onto a quartz substrate. Inset shows a plot of/λversus 1/λto determine the optical bandgap of the GO sheet. (k,l) HR XPS C 1 s (k) and O 1 s (l) line scans of GO that was grown on Cu at 240 °C for 120 min. (m) Grazing-angle FT-IR spectrum of a six-layer-stacked GO that was grown on Cu at 240 °C for 120 min and then transferred onto an atomically flat, clean surface of Au film deposited on SiO2/Si. Synthesis of the GO sheets We developed a solution-free, physical synthesis process for the synthesis of monolithic chemically modified C sheets on Cu surfaces that relies on a diffusion-assisted synthesis (DAS) approach [14] , as shown in Figure 1a . Initially, 1-μm-thick polycrystalline Cu foils were used; these Cu foils exhibited strong rolling features with irregular grain structures that were produced during the manufacturing process [15] ( Supplementary Fig. 1a ). In the annealing step, the Cu foils were annealed at ∼ 790 °C in ambient hydrogen to yield a strong (111) texture with aligned grain boundaries (GBs) normal to the foil surface and 30–50-μm-sized grains with smooth surfaces ( Supplementary Fig. 1b ). The morphology, crystallinity and distribution of atomic impurities in the Cu foils before and after the annealing process are presented in Supplementary Fig. 1 . Next, the annealed Cu foils were physically attached onto a SiO 2 /Si substrate and were covered with graphite powder that acts as a solid C source. The C–Cu–substrate assembly, which was clamped at a pressure of ∼ 1 MPa, was then placed in a quartz tube under a flow of argon gas at atmospheric pressure and heated up to 260 °C for 5–120 min. After the solid C source was removed, the samples were cleaned and the Cu foils were detached from the substrate ( Supplementary Methods ). It is worth noting that we always observed the formation of a monolithic graphene framework on the reverse side of the Cu foils, rather than on the surface of the SiO 2 /Si substrate. Figure 1b–e shows typical optical microscopy images of the annealed, bare Cu foils and the as-synthesized graphene frameworks on the reverse side of the Cu foils before and after oxidation in air at 200 °C for 120 min. The resulting graphene framework was found to be highly resistant to oxidation, thus indicating the presence of a monolithic form of C sheets on the Cu surface [16] . The hexagonal configuration of the graphene framework in the samples was evidenced by plan-view transmission electron microscopy (TEM; Fig. 1f,g ). Figure 1: Structural and optical characterization of monolithic GO sheets on Cu. ( a ) Schematic representation of the modified DAS process for obtaining monolithic GO sheets on the reverse side of a Cu foil. This process includes the elementary steps in the DAS process: the annealing of the Cu foil; the physical attachment of the Cu foil onto the substrate and the preparation of the C–Cu–substrate diffusion couple; heating of the assembly in ambient argon (below 260 °C) and the formation of monolithic GO sheets at the Cu/substrate interface; and the detachment of the Cu foils after removal of the solid C sources from the foil surface. ( b – e ) Optical microscopy images of annealed Cu foils ( b , d ) and GO-covered Cu foils ( c , e ) before ( b , c ) and after ( d , e ) oxidation in air at 200 °C for 120 min (scale bars, 150 μm). ( f , g ) A bright-field TEM image of the GO sheet (scale bar, 1 μm) ( f ) and its corresponding selected area electron diffraction pattern (scale bar, 5 nm −1 ). ( g ) Most micro-crystallites were polycrystalline. ( h ) Representative Raman spectra of GO that was grown on a Cu surface at 240 °C for 60 min (bottom) and 120 min (top), and then transferred onto SiO 2 (300 nm)/Si. ( i ) Raman map of the G/2D bands (top) and the FWHM of the 2D band (bottom) of GO that was grown on Cu at 240 °C for 60 min and then transferred onto SiO 2 (300 nm)/Si (scale bars, 10 μm). ( j ) Optical transmittance of GO that was grown on Cu at 240 °C for 120 min and then transferred onto a quartz substrate. Inset shows a plot of / λ versus 1/ λ to determine the optical bandgap of the GO sheet. ( k , l ) HR XPS C 1 s ( k ) and O 1 s ( l ) line scans of GO that was grown on Cu at 240 °C for 120 min. ( m ) Grazing-angle FT-IR spectrum of a six-layer-stacked GO that was grown on Cu at 240 °C for 120 min and then transferred onto an atomically flat, clean surface of Au film deposited on SiO 2 /Si. Full size image Figure 1h shows representative Raman spectra of samples that were obtained at a temperature of 240 °C for 60–120 min and then transferred onto SiO 2 /Si(100). These spectra indicate the significant presence of foreign species in the graphene framework. The spectra for all of the samples exhibit three primary features: a D band at ∼ 1,348 cm −1 , a G band at ∼ 1,592 cm −1 and a 2D band at ∼ 2,687 cm −1 , which are all typical peak positions for graphene [14] , [16] , [17] , [18] , [19] , [20] , [21] . However, the Raman spectra of the samples consistently show an intense D band ( I D / I G ≥1.0) related to domain boundaries, impurities and growth-nucleation sites [22] , [23] , [24] , [25] . Based on the Tuinstra–Koenig relationship [26] , the average distance between the defects in our samples was estimated to be less than ∼ 19 nm. The associated G/2D band and the full-width at half-maximum (FWHM) of the 2D band maps, as shown in Fig. 1i , illustrate the uniformity of the samples over a large area (70 μm × 70 μm). The samples primarily consisted of a single-layer graphene framework (as identified by I G / I 2D ≤0.4 and a FWHM of the 2D band of ∼ 38 cm −1 ) and bi- and multi-layered regions that resembled ridge structures [14] akin to GBs in the annealed Cu foils. The graphene framework seems to be predominantly composed of a single layer when analysed using Raman spectra and maps. Interestingly, the formation of a graphene framework on Cu appears to have been self-limited; growth that proceeded for 120 min yielded a single-layer structure similar to that obtained following 60-min growth based on the Raman structure. The optical transmittance of the samples that were grown for 120 min decreased by 2.3–2.5% ( Fig. 1j ), thus implying that the average thickness of these samples corresponded approximately to that of a monolayer [27] . In contrast to pristine graphene that has no bandgap [17] , [18] , [19] , however, the optical bandgaps of the graphene frameworks that were transferred onto quartz were measured to be ∼ 2.21 eV, based on UV–vis spectroscopy ( Fig. 1j , inset), suggesting the presence of foreign species in the graphene framework [28] , [29] . Furthermore, atomic force microscopy (AFM) measurements show that the surface root-mean-square roughness of the graphene frameworks that were transferred onto SiO 2 /Si(100) was 2–3 times larger than that of the pristine graphene on SiO 2 /Si(100), which could be attributed to the random covalent attachment of foreign species onto the surface of the graphene framework [30] . We therefore further investigated the presence and chemical states of foreign species in the samples using X-ray photoelectron spectroscopy (XPS) and Fourier transform-infrared (FT-IR) spectroscopy. Typical XPS wide-scan survey spectrum of the samples shows substantial C1s and O1s peaks at ∼ 284.4 and 530.4 eV, respectively ( Supplementary Fig. 2a ). A high-resolution (HR) C1s line-scan spectrum exhibited a dominant peak at ∼ 284.4 eV, which corresponds to the graphite-like sp 2 -hybridized C ( Fig. 1k ), thus indicating that most of the C atoms formed a 2D honeycomb backbone structure. Two additional peaks are located at ∼ 285.3 and 288.0 eV, which could be attributed to oxygenated groups [8] , [9] , [10] , [11] . The detailed chemical states of the oxygen functionalities on the samples can be witnessed by a HR O1s line-scan spectrum ( Fig. 1l and Supplementary Fig. 3 ). Grazing-angle reflectance FT-IR spectra of the samples further support the XPS results that there exist various oxygen functionalities in the graphene framework, including the vibration modes of hydroxyl, epoxide, carboxyl, carbonyl groups and sp 2 -hybridized C=C (in-plane vibrations) ( Fig. 1m ). On the basis of structural and optical characterizations, we concluded that the as-synthesized samples were highly ordered, predominantly monolayer GO sheets. Atomic structure of the GO sheets Next, we performed a closer examination of the structure of the GO sheets. 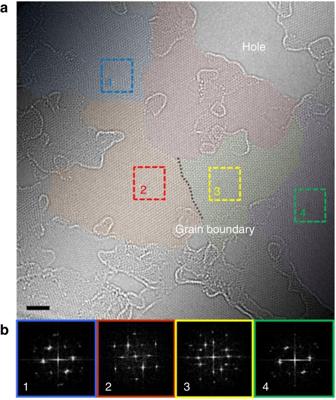Figure 2: Atomic structure of a GO sheet. (a) Atomic resolution, plan-view TEM image of a GO sheet that was grown on a Cu surface at 240 °C for 120 min and then transferred onto a TEM grid. The colour scheme highlights the different crystalline structures of the GO grains. Holes are observed after the transfer process of the GO sheet onto a TEM grid (scale bar, 2 nm). (b) FFT patterns of the regions specified ina. Figure 2a presents a typical HR-TEM image that was obtained using aberration-corrected instruments; the highly graphitic nature of our GO samples was in striking contrast to the structure of chemically synthesized GO [8] , [31] . The structure of our samples consisted of a highly ordered honeycomb lattice with a grain size of ∼ 10 nm, consistent with the value predicted from the Tuinstra–Koenig equation. The graphitic grains were mis-tilted along the azimuthal direction with respect to each other, and the interiors of the graphitic grains were found to be highly crystalline. Four typical fast FT (FFTs) of the HR-TEM image are illustrated in Fig. 2b , which together confirm the graphitic nature of the discrete grains. The presence of a significant amount of oxygen in our samples was further confirmed by electron energy loss spectroscopy in TEM ( Supplementary Fig. 2b ). The large graphitic area in the GO surface supports our hypothesis that the parent GO consists of a honeycomb lattice that is decorated with oxygenated functionalities. Bi- and multi-layer (≤4 layers) regions, which could be attributed to the ridge structures [14] , were frequently detected by HR-TEM. Both regions displayed distinct Moiré patterns that were caused by the stacking of individual hexagonal graphitic layers with different orientations [32] . Figure 2: Atomic structure of a GO sheet. ( a ) Atomic resolution, plan-view TEM image of a GO sheet that was grown on a Cu surface at 240 °C for 120 min and then transferred onto a TEM grid. The colour scheme highlights the different crystalline structures of the GO grains. Holes are observed after the transfer process of the GO sheet onto a TEM grid (scale bar, 2 nm). ( b ) FFT patterns of the regions specified in a . Full size image Existence of an incubation time in GO synthesis We grew GO sheets for various periods under isothermal conditions. For growth times of <60 min at 240 °C, the Raman spectra indicate that the as-synthesized films contained a mixture of disordered and graphitic C areas, and that the relative surface coverage between disordered and graphitic C showed a critical dependence on the growth time, as shown in Fig. 3a . The resulting film was predominantly a disordered C layer with >95 % surface coverage after 5 min of growth ( Fig. 3b ). However, the surface coverage of the graphitic C layer increased linearly from ∼ 30 to 100 % as growth time increased from 5 to 60 min, thus revealing the existence of an incubation time for graphitic C growth on Cu at low temperatures. 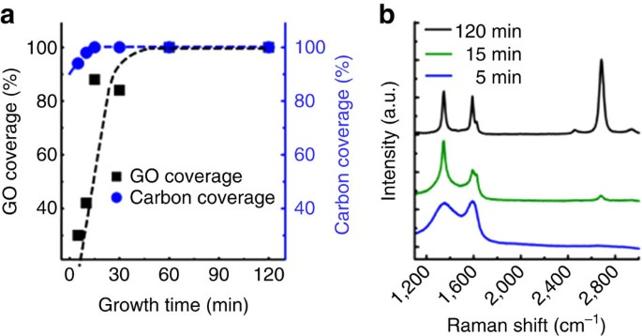Figure 3: Formation of a monolithic GO sheet on a Cu surface with various incubation times. (a) Plot of GO coverage (black squares) and C-segment coverage (blue circles) on a Cu surface as a function of growth time at 240 °C based on the Raman structure. (b) Comparison of the Raman spectra of GO sheets that were grown on Cu at 240 °C for 5 min (blue), 15 min (green) and 120 min (black), and then transferred onto a SiO2(300 nm)/Si substrate. Figure 3: Formation of a monolithic GO sheet on a Cu surface with various incubation times. ( a ) Plot of GO coverage (black squares) and C-segment coverage (blue circles) on a Cu surface as a function of growth time at 240 °C based on the Raman structure. ( b ) Comparison of the Raman spectra of GO sheets that were grown on Cu at 240 °C for 5 min (blue), 15 min (green) and 120 min (black), and then transferred onto a SiO 2 (300 nm)/Si substrate. Full size image Mechanism for the formation of GO sheets A key question is why the GO sheets form through the DAS process using solid C at low temperatures. Central to this issue are the origin of O atoms in the resulting graphene framework and the diffusion of C and O atoms through the Cu foil, followed by the formation of the GO sheets on a Cu surface after an incubation period. 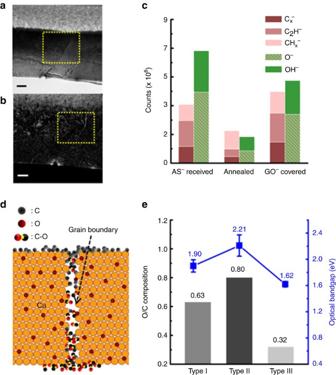Figure 4: Origin of the C and O atoms and controllable O/C composition and bandgap energy in the GO sheets. (a,b) Zero-loss filtered bright-field cross-sectional TEM image (a) of the Cu foil after DAS at 240 °C for 120 min (using an energy slit width of 10 eV to select the zero-loss peak) and the corresponding C map (b). The yellow rectangles denote the same location in the TEM images (scale bars, 0.2 μm). (c) Changes in the elemental composition of C−and O−containing species, based on TOF-SIMS analysis of the surfaces of an as-received Cu foil, an annealed Cu foil at 790 °C in ambient hydrogen, and a GO-covered Cu foil that was grown at 240 °C for 120 min. (d) Schematic diagram of GO growth mechanism during DAS process using solid C; C atoms began to diffuse through the Cu along the GBs of the foil while trapping the O species dissolved in the Cu, leading to the predominant diffusion of C–O molecules over Cu as well as through GBs. (e) Changes in the O/C composition and the calculated bandgap energy in the GO sheets that were formed on a Cu surface under three different conditions. The GO sheets were synthesized at 240 °C for 60 min with the Cu foil annealed at 790 °C for 20 min (type I); at 240 °C for 120 min with the Cu foil annealed at 790 °C for 20 min (type II); and at 240 °C for 120 min with the Cu foil annealed at 790 °C for 260 min (type III). Error bars are the standard deviation of the bandgap energy measured in five different samples grown under the same condition. Figure 4a,b displays a representative zero-loss energy-filtered bright-field TEM image and a corresponding elemental map of C (based on the three-window technique [33] ) of the Cu foil following DAS process at 240 °C for 120 min. The predominant presence of C atoms along the GBs in the Cu is clearly visible from the elemental map; therefore, it can be stated that the GBs are the dominant diffusion pathway for C atoms during the DAS process. After the C atoms diffuse to the reverse side of the Cu foil, nucleation results from competition between the surface-diffusion processes, followed by capture of the supercritical nucleus and the evaporation of C-adatoms from the Cu surface. Considering the high activation energy ( ∼ 6 eV (ref. 34 )) for the desorption of C-adatoms and the very low activation energy ( Table 1 ) of C-adatom diffusion on Cu, we suggest that the formation of the graphene framework on Cu can be described by C attachment/detachment to the edges of the nuclei as the rate-limiting step at low temperatures, thus resulting in the occurrence of two growth regimes ( Fig. 3a ). Figure 4: Origin of the C and O atoms and controllable O/C composition and bandgap energy in the GO sheets. ( a , b ) Zero-loss filtered bright-field cross-sectional TEM image ( a ) of the Cu foil after DAS at 240 °C for 120 min (using an energy slit width of 10 eV to select the zero-loss peak) and the corresponding C map ( b ). The yellow rectangles denote the same location in the TEM images (scale bars, 0.2 μm). ( c ) Changes in the elemental composition of C − and O − containing species, based on TOF-SIMS analysis of the surfaces of an as-received Cu foil, an annealed Cu foil at 790 °C in ambient hydrogen, and a GO-covered Cu foil that was grown at 240 °C for 120 min. ( d ) Schematic diagram of GO growth mechanism during DAS process using solid C; C atoms began to diffuse through the Cu along the GBs of the foil while trapping the O species dissolved in the Cu, leading to the predominant diffusion of C–O molecules over Cu as well as through GBs. ( e ) Changes in the O/C composition and the calculated bandgap energy in the GO sheets that were formed on a Cu surface under three different conditions. The GO sheets were synthesized at 240 °C for 60 min with the Cu foil annealed at 790 °C for 20 min (type I); at 240 °C for 120 min with the Cu foil annealed at 790 °C for 20 min (type II); and at 240 °C for 120 min with the Cu foil annealed at 790 °C for 260 min (type III). Error bars are the standard deviation of the bandgap energy measured in five different samples grown under the same condition. Full size image Table 1 Calculated activation energy barriers (in eV) of the correlated diffusion of C- and O-containing precursors on Cu(111) and Cu(100) surfaces. Full size table To elucidate the origin of the O atoms, we performed time-of-flight secondary ion mass spectroscopy (TOF-SIMS) on three different samples. Figure 4c shows the relative change in the intensities of C − and O − containing species that were ejected from (a) an as-received Cu surface, (b) a Cu surface annealed at ∼ 790 °C in ambient hydrogen, and (c) a GO-covered Cu surface after DAS process at 240 °C for 120 min. The levels of oxygen and oxidizing elements on the Cu surface increased as a result of the DAS process, and there was also an increased level of C-containing compounds, owing to C-adatom diffusion along the GBs in the Cu. Considering that we found the O distribution with an annealed Cu foil to be quite uniform (based on energy-dispersive spectroscopy ( Supplementary Fig. 1b ) in TEM), and given that DAS was conducted in an inert ambient, we suggest that there was no driving force for spontaneous O diffusion through the Cu lattices or along the GBs. In addition, the residual O atoms on the Cu surface cannot have diffused into the graphitic lattice during the DAS process, because O atoms have a higher affinity for the Cu surface than C atoms [35] and our synthesis was conducted at low temperatures. Therefore, we inferred that the O atoms in the resulting GO sheets have diffused from the interior of the Cu crystals during the DAS process. We performed spin-polarized density functional theory (DFT) calculations [36] , [37] to investigate the mechanism of the C- and O-diffusion processes that are associated with the formation of GO on the reverse side of the Cu foils. Here, the diffusion processes of monomers, dimers and trimers, including C- and O-adatoms, were considered on Cu(111) and Cu(100) surfaces, because the activation energy barrier of the correlated diffusion of multi-adatoms on metal surfaces generally increases with the number of adparticles [38] . The DFT calculation results are summarized in Table 1 (details of the calculations are presented in Methods section). We note that the lowest energy barriers for the diffusion of C- and O-adatoms were achieved when C–O dimers diffused over Cu, irrespective of the orientation of the crystallographic plane. The energy barriers of C–O dimers on Cu(111) and Cu(100) surfaces were 0.105 and 0.188 eV, respectively. This finding indicates that the O atoms at the GBs in Cu preferentially combined with the diffusing C atoms with a dangling bond, followed by the diffusion of C–O molecules over Cu as well as through GBs ( Fig. 4d ). Considering very high tracer diffusion coefficients ( D t ) (details of the calculations are presented in Methods section), C-containing precursors reaching the reverse side of the Cu foil diffuse laterally along the Cu(111) surface for a short period and lead to the growth of a graphene framework over large areas after an incubation time, driven by the strong affinity of C atoms to self-assemble and expand the sp 2 lattice [39] . Considering that C–C and C–O bonds tend to segregate and that O atoms are almost insoluble in C clusters at low temperatures [10] , [40] , the resulting films become highly graphitic sheets that are decorated with oxygenated functionalities. Control of O/C composition and tunable bandgap energy The O content in the GO sheets directly correlates with the heating profile of the Cu foil during the annealing step. Modifying the heating profile enables the residual O concentration in Cu to be controlled; therefore, it is easy to tune the composition of O atoms in the resulting GO sheets. GO becomes less oxygenated as the heating proceeds; for example, the O/C composition in GO was decreased from 0.80 to 0.32 as the annealing time increased from 20 to 260 min at ∼ 790 °C ( Fig. 4e and Supplementary Fig. 4 ). This result is remarkable because the precise control of O content in GO during the synthesis has not yet been reported for any chemical synthesis processes [8] , [9] , [10] , [11] . Importantly, the bandgap energy of GO can be controlled by varying the O/C composition. UV–vis measurements show that the bandgap of GO decreases from ∼ 2.2 to 1.6 eV as the O/C composition decreases from 0.80 to 0.32 ( Fig. 4e ). This result demonstrates the ability to control the bandgap of GO by simply annealing the Cu foil before solid-state diffusion. It is worthwhile to note that the average sizes of graphitic grains in the GO sheets were all ∼ 10 nm using HR-TEM measurements, regardless of O/C composition. However, we have found the systematic variations of the bandgap values of the GO sheets by varying the O/C composition, suggesting that the oxygen functionalities existing on the graphitic grains in GO are the cause of bandgap tunability. In principle, the bandgap can be further reduced by long-period thermal annealing of the Cu foil. Tunable electronic properties of the GO sheets The electronic properties of the individual GO sheets with the different O/C compositions were measured via back-gated GO-based FET devices. FET devices with a channel length of 5 μm and channel widths of 200 μm (O/C ∼ 0.8) and 20 μm (O/C ∼ 0.3) atop 300 nm SiO 2 with a p-Si back gate fabricated by the conventional photolithography. All of the reported electrical measurements were taken under vacuum at temperatures ranging from 20 to 300 K. As shown in Fig. 5a,b , irrespective of the O content in the GO, the ‘V’ shape of the ambipolar transfer characteristics and the shift of minimum conduction point to positive gate voltage are observed for both samples, which are characteristics that are normally observed in both prinstine graphene [41] and chemically reduced GO [8] , [9] , [10] , [11] . The principal similarity between the gate dependence of the GO sheet and graphene is a direct indication of the presence of intact graphitic grains in the GO sheets [42] , as observed in HR-TEM and Raman results of the GO. It was found that achieving lower O/C composition yields significantly enhanced electrical performance and the GO sheets exhibited tunable field-effect mobilities from 19.7±4.1 to 82.6±10.2 cm 2 V −1 s −1 at room temperature as the O/C composition decreased from 0.80 to 0.32. We note that the as-synthesized GO sheets were electrically active without any further chemical and/or thermal treatment, in contrast to chemically derived GO [8] , [9] , [10] , [11] , and the measured carrier (hole) mobility of the GO sheet with O/C composition of 0.32 is superior to the previously reported mobility values of chemically reduced GO-based FETs [1] , [42] , [43] , [44] . The higher overall mobilities in our devices, compared with those achieved in chemically reduced GO flakes, could be attributed to the morphological nature of the monolithic GO sheets without any junction/overlapping regions between graphitic grains since the weak coupling between adjacent GO flakes (that is, the high internanosheet resistance) may cause the device performance to be much less than that of single nanosheets [45] . In addition, the conductivity of both samples at all gate voltages from −80 to +80 V increased with temperature, indicating that both types exhibit semiconducting behaviour, in contrast to the semimetallic prinstine graphene [41] . 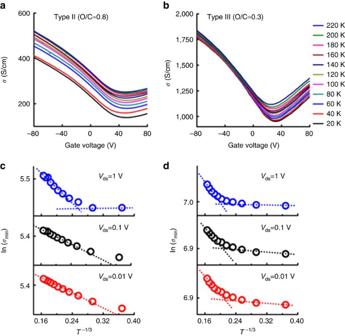Figure 5: Tunable electrical properties of the GO sheets with varying the O/C composition. (a,b) Transfer characteristics of the GO sheets with different O/C compositions of 0.80 (type II,a) and 0.32 (type III,b) measured at temperatures ranging from 20 to 300 K (Vds=0.01 V). (c,d) Minimum conductivityσminof the GO sheets with different O/C compositions of 0.80 (type II,c) and 0.32 (type III,d) at three different values of bias voltage (Vds) ranging from 0.01 to 1 V as a function ofT−1/3. Figure 5: Tunable electrical properties of the GO sheets with varying the O/C composition. ( a , b ) Transfer characteristics of the GO sheets with different O/C compositions of 0.80 (type II, a ) and 0.32 (type III, b ) measured at temperatures ranging from 20 to 300 K ( V ds =0.01 V). ( c , d ) Minimum conductivity σ min of the GO sheets with different O/C compositions of 0.80 (type II, c ) and 0.32 (type III, d ) at three different values of bias voltage ( V ds ) ranging from 0.01 to 1 V as a function of T −1/3 . Full size image To further investigate the conduction mechanism in our monolithic GO sheets, we examined the variation of the conductivity at minimum conduction point ( σ min ) as a function of T −1/3 for three different values of bias voltage ( V ds ), as shown in Fig. 5c,d . In the case of the GO sheet with a higher O/C composition of 0.80, the best linear fits of the temperature-dependent data were obtained at all examined V ds by plotting ln( σ min ) versus T −1/3 , pointing toward 2D variable-range hopping (2D-VRH) as a plausible charge transport mechanism [42] , [46] , whereas deviation from the 2D-VRH model was observed at the lower temperature regime for the highest value of bias voltage ( V ds =1 V). In view of the above-described structural measurements, that is, HR-TEM and Raman results of the GO, hopping presumably occurs between the intact graphitic grains, which are separated by clusters of atomic defects. The deviation from linear fit at the lower temperautre regime can be explained by the contribution of the field-driven conduction without thermal activation [46] , [47] , [48] . However, the GO sheet with a lower O/C composition of 0.32 showed a deviation from the linear fit (that is, 2D-VRH model) at all examined V ds and the temperature dependence of the σ min at the higher temperature regime can be fitted reasonably well with the Arrhenius model, suggesting that thermally excited carriers begin to dominate electrical conduction [49] . Based on the transport properties of the GO sheets, we can conjecture that the bandgap energy of GO was narrowed down as the O/C composition decreased from 0.80 to 0.32, which is in agreement with the UV–vis measurement. Overall, a clear trend is observed between variations in the O/C composition and the optoelectronic properties of the resulting GO sheets. By monitoring optoelectronic properties, we have found that the electrical transport mechanism in our physically synthesized, monolithic GO sheets is, despite the significantly higher conductivity, more similar to chemically reduced GO than to as-synthesized, chemically derived GO. Our finding suggests that highly tunable GO sheets may enable the design of monolithic semiconducting and optoelectronic devices, in combination with our solution-free, physical synthesis approach. We have demonstrated a new physical method for the controllable growth of monolithic GO sheets on Cu surfaces at low temperatures. This technique offers a more promising approach to the precision assembly of graphene-based devices than established chemical syntheses and could complement existing production techniques. The simplicity of solution-free, physical synthesis of the GO sheets in combination with tunable electronic and optoelectronic properties may provide the shortest path to precision device assembly based on graphene and its derivatives. Furthermore, our physical method can pave the way for the realization of monolithic, 2D chemically modified C sheets with tunable composition, which are produced by pre-treating the metallic foils (and/or films) under various conditions (ambient, temperature, doping and so on) before the DAS process. Considering the inherent potential of 2D C sheets with high flexibility, transparency and mechanical strength, one could anticipate the use of stacked heterostructure based on 2D sheet designs for the next generation of flexible nanodevices. Finally, advances in the development of ultrahigh-purity metallic diffusion media with a controlled doping concentration can open the door to the realization of graphene sheets with a defined substitutional doping concentration. Synthesis of monolithic GO sheets on Cu foil via DAS First polycrystalline Cu foil (99.97% purity, 1-μm thickness, Good Fellow, cut to 1 cm × 1 cm) was transferred to an ultrahigh vacuum (UHV) chamber system (base pressure ∼ 1 × 10 −10 Torr) and was annealed at ∼ 790 °C for 20–260 min in ambient hydrogen (99.9999% purity, pressure ∼ 1 × 10 −6 Torr). In the UHV system, the substrate temperature was measured using a k-type thermocouple that was directly connected to the substrate susceptor before annealing experiments; accuracy was ±5 °C. Variations in the annealing time allowed the O content in the Cu foil to be tuned. Next the Cu foil was placed onto a SiO 2 /Si substrate and the Cu foil was coated with graphite powder (Aldrich, product number 496596), then the graphite powder was pressed onto the Cu surface. At temperatures below 260 °C, C in the samples began to diffuse through the Cu along the GBs of the foil while trapping the O species dissolved in the Cu. The substrate temperature was measured using a k-type thermocouple that was directly connected to the molybdenum sample holder; accuracy was ±10 °C. As the diffusing C and O atoms reached the reverse side of the Cu foil, they created a thin film of GO over the incubation time. The pressure promotes the movement of C through the Cu foil. Further details are given in the Supplementary Methods . We note that 1-μm-thick Cu foil provides the optimum process efficiency for the DAS process among commercially available Cu foils with thicknesses ranging from 0.5 to 50 μm. Foils that are thinner than 1 μm exhibit shorter durations with easier control over the DAS process, although there is a trade off in the ease of sample handling. Transfer process of GO sheets Poly(methyl methacrylate) (PMMA) was spin-coated onto the GO-grown Cu foils at 4,000 r.p.m. for 20 s. The Cu foils were etched in an aqueous solution of (NH 3 ) 3 S 2 O 8 . After being rinsed in deionized water for 30 min, the PMMA-coated GO was transferred onto the target substrate. Then the sample was dried on a hot plate at ∼ 80 °C for 10 min. Finally, the PMMA was removed by washing with acetone. Atomic force microscopy The surface morphologies of the as-received, annealed and GO-covered Cu foils were observed using an AFM (Veeco Multimode V) operating in tapping mode. The surface root-mean-square roughness of the samples was estimated from over 20 different regions per sample, with a scan size of 5 μm × 5 μm. Raman spectroscopy and mapping The presence of a highly ordered graphene framework was confirmed by Raman spectroscopy. Both the Raman spectra and maps were collected from a graphene framework that had been transferred onto a 300-nm-thick SiO 2 layer on Si. The Raman spectroscopy and mapping were carried out on a WiTec alpha 300R M-Raman system with a 532 nm excitation wavelength (2.33 eV); the laser spot had a dimension of ∼ 640 nm for a × 50 objective lens with numerical aperture of 0.5 and the laser power was ∼ 2 mW. The Raman spectra were analysed and Raman images were constructed using a computer-controlled x - y translation stage with a raster scan. A spectroscopic image was created by measuring the Raman spectrum of each individual pixel with a 70 μm × 70 μm step size using WiTec Project software. The Raman data presented in this manuscript, such as I G / I 2D and the FWHM values of the G and 2D bands, are arithmetical averages of values that were measured at more than 30 different points per sample. UV–vis spectroscopy The optical transmittance of a graphene framework that was transferred onto a quartz plate was measured using UV–vis spectroscopy (Varian, Cary 5000 model) between 200 and 800 nm in dual-beam mode. The optical band gap, as determined from the plot of / λ versus 1/ λ following Tauc’s equation [50] , is an arithmetic average of values that were measured for five different samples grown under the same condition. X-ray photoelectron spectroscopy The presence and chemical states of foreign species in the graphene framework were investigated using XPS. The XPS studies were conducted on a K-alpha spectrometer (Thermo Fisher) using aluminium Kα non-monochromatic X-ray excitation at a power of 72 W, with an analysis area diameter of ∼ 0.4 mm and a pass energy of 50 eV for the electron analysis. The base pressure of the analysis chamber was below ∼ 1 × 10 −9 mbar. The O/C compositions in the graphene frameworks were determined by dividing the individual peak areas in an XPS wide-scan survey spectrum, after appropriate background subtraction, by their respective atomic sensitivity factor. Fourier transform-infrared spectroscopy To investigate the special oxygen configuration in the gaphene framework, the reflectance FT-IR spectrum of a six-layer-stacked graphene framework that was transferred onto atomically flat, clean surface of Au film deposited on SiO 2 /Si was measured using the Agilent Cary 670 FTIR spectrometer interfaced to a Seagull accessory set for reflection analysis (with an incidence angle of 84°), a mercury cadmium telluride detector and a Ge on KBr beam splitter. To overcome the low throughput in incidence angle mode, six different samples grown under the same condition were mechanically stacked onto Au surface. Time-of-flight secondary ion mass spectroscopy To compare the elemental compositions of C and O atoms in the as-received and annealed Cu foils before and after the DAS process, TOF-SIMS measurements were carried out on an ION-TOF (Münster, Germany) instrument. A pulsed 25 keV Bi + primary ion source (average current: 1.0 pA; pulse width: 12.1 ns; and repetition rate 100 μHz) was used over a 500 μm × 500 μm area at an operating pressure of ∼ 1 × 10 −9 mbar. Negative-ion profiles were recorded and analysed; this technique is ideally suited to searching for possible correlations related to the ejected secondary ion polarity of C and O atoms [51] . Cross-sectional TEM of Cu foils and GO/Cu foils The TEM samples were prepared as follows: the two surfaces of Cu foil were glued together with a Si substrate to support the flexible 1-μm-thick Cu foils. This Si-sandwiched Cu foil was sliced into 2-mm-thick pieces by using a low-speed diamond saw. After being polished to a residual thickness of ∼ 10 μm, the sample was finally milled by an Ar + ion-beam (PIPS, Gatan Inc.). Substantial heating of the TEM foils and, consequently, the introduction of artefacts were avoided by means of double-sided ion-beam etching at small angles (<6°) and low-etching energies (acceleration voltage 2.5 kV; beam current <8 μA) with liquid-nitrogen cooling ( ∼ 150 K; ref. 52 ). For energy-filtering TEM imaging, a Tecnai F20 microscope (installed at Seoul National University) that was operating at 200 kV and equipped with a Gatan image filter system was used. The Digital Micrograph software (Gatan Inc.) was used for the image processing and analysis. HR plan-view TEM of the GO sheets Using a direct transfer method [53] , the GO sheets were transferred onto Quantifoil TEM grids. However, after the transfer process onto a TEM grid, we frequently observed the formation of ∼ 10–100-nm-sized holes in the GO sheets. HR-TEM images and the corresponding FFT patterns of the GO sheets were obtained on an FEI Titan cube G2 60–300 at UNIST, which was equipped with an image-aberration corrector and monochromator. The microscope was operated at an accelerating voltage of 80 kV to decrease beam damage to the GO sheets. FET device fabrication and electrical characterizations Bottom-gated FET devices were fabricated by transferring the GO sheets onto p-Si substrates with 300 nm thermal oxide. p-Si was used as the gate electrode. FET devices with a channel length of 5 μm and channel widths of 200 μm (O/C ∼ 0.8) and 20 μm (O/C ∼ 0.3) were fabricated by conventional photolithography and the O 2 plasma-etching process. We used a larger channel width in the sample with O/C composition of 0.80 to make a clear distiction between source-drain current values owing to the lower conductivity of the sample. Source-drain electrodes (Cr/Au: 10 nm/60 nm) were deposited by using an e-beam evaporator. The measurements of transport characteristics were conducted with a cryogenic probe station (Lake Shore, CRX-4K) at temperatures from 20 to 300 K. Before measurements, we put the samples into a vacuum chamber of ∼ 1 × 10 −6 Torr for 24 h to reduce the adsorbed impurity molecules, such as water vapours, on the GO sheets and then cooled down the sample temperature. From the plot of the source-drain current as a function of gate voltage from −80 to 80 V, we extracted carrier mobility values from the slope. At each temperature, the conductivity values were calculated by using an average thickness of 1 nm for our GO sheets, which was obtained from our AFM studies. DFT calculations All calculations considered the spin-polarized DFT [36] , [37] . We calculated the transitional state (TS) energy of a monomer, dimer and trimer diffusion of C- and O-adatoms on both Cu(111) and Cu(100) surfaces. The framework of TS energy calculation for atomic and molecular diffusion was based on refs 14 , 54 . The calculations were conducted by using the CASTEP module in Materials Studio 6.1 that provides various modelling and simulation environment for atomic and molecular structure determination, property prediction or simulation method in material science and chemistry. The CASTEP is a full-featured materials modelling code based on a first-principles quantum mechanical description of electrons and nuclei of atoms and molecules. It uses the robust methods of a plan wave basis set and pseudopotentials. The ultrasoft pseudopotentials [55] and the generalized gradient approximation were used with the exchange-correlation functional of Perdew et al. [56] Monkhost and Pack [57] k-point mesh was 3 × 3 × 1 that was used to test the Brillouin zone in the reciprocal space and the fine accuracy option was adapted for all calculations. Five layers of atomic plane filled with Cu atoms were used to simulate the Cu(111) and Cu(100) surfaces. Supplementary Fig. 5 shows the typical atomic structure model that was constructed for atomic and molecular diffusion on Cu consisted of 32 atoms with periodic boundary conditions along the in-plane directions. The lattice constant of atomic structure is 3.615 Å in both Cu(111) and Cu(100). To find TS energy diagram, we ran the calculation by CASTEP with a single linear synchronous transit, followed by repeated conjugate gradient minimizations and quadratic synchronous transit maximization until a transition state had been located. Before the TS search calculation, all models had relaxation to have most stable state. Supplementary Fig. 6 shows the diagram of calculated TS energy of atomic or molecular diffusion on Cu(111) surface: C monomer, C dimer, O monomer, O dimer and C–O molecules. From Supplementary Fig. 6a , it is seen that the calculated barrier energy of C monomer diffusion on the Cu(111) surface is 0.223 eV, whereas that of C dimer is 0.454 eV. For O diffusion, the barrier energies of minimum diffusion pathway for an O monomer as well as O dimer on Cu(111) are 0.295 and 0.485 eV, respectively, as shown in Supplementary Fig. 6b . In case of both CO and C 2 O molecular diffusion on Cu(111) surface, the calculated barrier energies are 0.105 and 0.633 eV, respectively, as represented in Supplementary Fig. 6c . Same calculation was repeated for Cu(100) surface, and Supplementary Fig. 7 shows the diagram of calculated TS energy of atomic or molecular diffusion on Cu(100) surface. As shown in Supplementary Fig. 7a , the calculated barrier energies of diffusion are 2.118 and 0.883 eV for C monomer and C dimer, respectively. From Supplementary Fig. 7b , it is known that the calculated barrier energy of an O monomer diffusion on Cu(100) surface is 0.940 eV, whereas that of O dimer is 1.121 eV. As represented in Supplementary Fig. 7c , the calculated barrier energies of a CO and a C 2 O molecule diffusion on Cu(100) surface are 0.188 and 0.595 eV, respectively. All results of calculation are summarized in Table 1 . The result of calculation performed in this study shows the different diffusion behaviour between C and O on the Cu(111) as well as Cu(100) surfaces. Comparing the diffusion behaviour of C and O on Cu(111) surface, the barrier energy of C diffusion increases as the diffusional species changes from monomer (0.223 eV) to dimer (0.454 eV), also O shows the increase in the barrier energy of diffusion when it changes from monomer (0.295 eV) to dimer (0.485 eV). In case of diffusion on Cu(100), the results of C show the trend to oppose to that of Cu(111). That is, the barrier energy of C diffusion decreases as the diffusional species changes from monomer (2.118 eV) to dimer (0.883 eV). But O shows increase in the barrier energy of diffusion when it changes from monomer (0.940 eV) to dimer (1.121 eV) as same with that of Cu(111). In all cases, however, the lowest barrier energy of diffusion can be achieved when the C–O molecule diffuses on Cu surface irrespective of crystallographic plane, compared with those of C and O, that is, the barrier energies of diffusion of C–O molecule are 0.105 eV on the Cu(111) and 0.188 eV on the Cu(100), respectively. To examine the diffusion of C-containing precursors reaching the reverse side of the Cu foil, we have calculated the tracer diffusion coefficients ( D t ) of both C monomer and C–O molecule along the Cu(111) surface. The hopping rates of C monomer and C–O molecule can be found by the Arrhenius equation Γ=Γ 0 exp(− E b / kT ), which results in room temperature hopping rates of ∼ 1.70 × 10 9 and 1.68 × 10 11 s −1 , respectively, with an attempt frequency of Γ 0 =1.0 × 10 13 Hz. In addition, the tracer diffusion coefficients of C monomer and C–O molecule can be expressed in terms of the hopping rate Γ and the mean square jump length ‹ l 2 ›: D t =Γ‹ l 2 ›/(2d), and are found to be ∼ 18.5 and 1,830 μ m 2 s −1 at room temperature using the lattice constant of Cu 3.615 Å, respectively. At T =240 °C, the tracer diffusion coefficients of C monomer and C–O molecule are expected to be ∼ 703 and 10,100 μ m 2 s −1 from our calculations, respectively. How to cite this article: Chu, J. H. et al. Monolithic graphene oxide sheets with controllable composition. Nat. Commun. 5:3383 doi: 10.1038/ncomms4383 (2014).